Triggers of key calcium signals during erythrocyte invasion byPlasmodium falciparum Invasion of erythrocytes by Plasmodium falciparum merozoites is a complex multi-step process mediated by specific interactions between host receptors and parasite ligands. Reticulocyte-binding protein homologues (RHs) and erythrocyte-binding-like (EBL) proteins are discharged from specialized organelles and used in early steps of invasion. Here we show that monoclonal antibodies against PfRH1 (an RH) block merozoite invasion by specifically inhibiting calcium signalling in the parasite, whereas invasion-inhibiting monoclonal antibodies targeting EBA175 (an EBL protein) have no effect on signalling. We further show that inhibition of this calcium signalling prevents EBA175 discharge and thereby formation of the junction between parasite and host cell. Our results indicate that PfRH1 has an initial sensing as well as signal transduction role that leads to the subsequent release of EBA175. They also provide new insights on how RH–host cell interactions lead to essential downstream signalling events in the parasite, suggesting new targets for malaria intervention. Plasmodium falciparum ( P. falciparum ) is the most virulent malaria parasite and accounts for the vast majority of deaths (WHO, http://www.rbm.who.int , 2010). Erythrocyte invasion is a complex multi-step process that is mediated by specific interactions between host receptors and parasite ligands. Junction formation between the merozoite and erythrocyte is a crucial step that allows the parasite to irreversibly bind to the host followed by the activation of its motor machinery system that drives the parasite completely into the erythrocyte [1] . Previous studies suggest the involvement of apical secretory organelles termed rhoptries and micronemes [2] . In Plasmodium species, a number of key parasite ligands that mediate critical interactions with host receptors during invasion are localized in these apical organelles [1] . Two protein families are used in early steps of invasion in P. falciparum : reticulocyte-binding protein homologues (RHs) and erythrocyte-binding-like proteins (EBLs) [3] . RHs and EBLs have been shown to have a crucial role in host cell recognition and sensing as well as virulence [4] . Members of both protein families can be found in all Plasmodium species, further highlighting their importance in malaria parasite biology. In EBLs, a duffy-binding-like (DBL) domain mediates specific binding to different host cell receptors [5] including glycophorins A, B and C as well as the Duffy blood group antigen [3] . In RHs, the precise erythrocyte-binding regions are still being delineated [4] , [6] , [7] , [8] , [9] , [10] , [11] , [12] , [13] ; complement receptor 1 (CR1) and basigin have been identified to be the receptors for PfRH4 (ref. 14 ) and PfRH5 (ref. 15 ), respectively. Although RHs have been proposed to have an early role in host cell sensing [16] , [17] , the EBLs are thought to have a direct role in junction formation [18] . This suggests that RH sensing and subsequent interaction with a suitable host erythrocyte sends a signal to the merozoite that triggers the subsequent steps of invasion [4] . Here we generate monoclonal antibodies (mAbs) against the erythrocyte-binding region RII-3 of PfRH1 (a member of the RH family in P. falciparum [7] ). We show that PfRH1 mAbs block merozoite invasion by specifically inhibiting calcium signalling in the parasite rather than by directly interfering with the erythrocyte binding of the parasite. We further show that the inhibition of this calcium signalling prevents EBA175 discharge and thereby prevents junction formation (a key step that enables the parasite to penetrate the erythrocyte using an actin-myosin motor [3] ). Our results demonstrate that PfRH1 and EBA175 have distinct functions, with PfRH1 having an initial sensing and signal transduction role that leads to subsequent EBA175 release from the microneme and to junction formation. These new insights might help to identify new targets for malaria intervention. Specific PfRH1 mAbs inhibit merozoite invasion In this work, we use PfRH1 to study key intracellular signalling events that lead to successful erythrocyte invasion. We have previously shown that antibodies targeting an erythrocyte-binding region (RII-3) of PfRH1 ( Fig. 1a ) can inhibit merozoite invasion [7] . Here we generated four monoclonal antibodies (mAbs: C49, C41, C2 and C50) against this region and validated their specificity using western blot and immunofluorescence assays. All antibodies recognize the expected 240- and 140-kDa-processed form of PfRH1 in T994 parasite culture supernatant, merozoite and schizont extracts, whereas no equivalent bands were detected in the PfRH1 knockout line T994ΔRH1 ( Supplementary Fig. S1a–c ). Immunofluorescence assays showed that all mAbs give punctuate patterns that are partially localized with EBA175 (a known microneme protein) at the apical end of merozoites in T994, consistent with the expected location of PfRH1 ( Supplementary Fig. S1d ). No staining was observed in T994ΔRH1 ( Supplementary Fig. S1e ), further confirming the specificity of the mAbs. 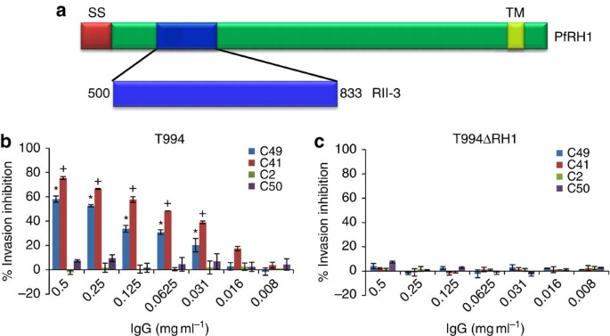Figure 1: Anti-PfRH1 mAbs significantly block parasite invasion. (a) Full-length PfRH1 including signal sequence (SS, red), erythrocyte-binding region RII-3 (blue, encompassing amino acids 500–833) and transmembrane domain (TM, yellow). (b,c) Invasion inhibition assays using anti-PfRH1 mAbs (IgG) in T994 (b) and T994ΔRH1 (c). Bar charts show mean±s.e.m.;n=3. *P≤0.0003 by one-way ANOVA, indicating that C49 successfully blocked the invasion in T994 compared with the invasion in the presence of C2 and C50.+P≤0.0003 by one-way ANOVA, indicating that C41 significantly inhibited the invasion compared with C2 and C50. Figure 1: Anti-PfRH1 mAbs significantly block parasite invasion. ( a ) Full-length PfRH1 including signal sequence (SS, red), erythrocyte-binding region RII-3 (blue, encompassing amino acids 500–833) and transmembrane domain (TM, yellow). ( b , c ) Invasion inhibition assays using anti-PfRH1 mAbs (IgG) in T994 ( b ) and T994ΔRH1 ( c ). Bar charts show mean±s.e.m. ; n =3. * P ≤0.0003 by one-way ANOVA, indicating that C49 successfully blocked the invasion in T994 compared with the invasion in the presence of C2 and C50. + P ≤0.0003 by one-way ANOVA, indicating that C41 significantly inhibited the invasion compared with C2 and C50. Full size image To establish whether the different mAbs were able to inhibit merozoite invasion, inhibition assays with increasing concentration of antibodies were carried out using T994 and T994ΔRH1 ( Fig. 1b,c ). We found that mAbs C2 and C50 have no significant effect on invasion, whereas both mAbs C49 and C41 inhibit invasion in a dose-dependent manner in T994. In contrast, none of the antibodies has any impact on T994ΔRH1, in line with their specificity to PfRH1. Similar results ( Supplementary Fig. S2a,b ) were obtained when using the parasite lines W2mef and W2mef/NM, which are known to differ in their requirement for PfRH1 in invasion [7] , [19] , suggesting that both C49 and C41 are invasion-inhibiting mAbs. To ensure that the invasion inhibitory effect is not because of the large size of the mAb (which could lead to a secondary blocking effect), we purified the Fab fragment of mAb C41 ( Supplementary Fig. S2c , insert) and performed invasion inhibition assays [20] , [21] . The purified C41 Fab fragment significantly blocks invasion in a dose-dependent manner in T994 parasites ( Supplementary Fig. S2c ), confirming that mAb C41 directly targets PfRH1. Inhibitory mAbs block invasion before junction formation Merozoite invasion inhibition by antibodies is often caused by antibodies directly interfering with the binding of the parasite to its receptor. We therefore assessed the ability of the different mAbs to inhibit PfRH1 binding to erythrocytes. Both non-inhibitory mAbs (C2 and C50) and inhibitory mAbs (C49 and C41), at concentrations (0.3 mg ml −1 ) shown to effectively inhibit merozoite invasion ( Fig. 1b ), have no impact on erythrocyte binding by PfRH1 ( Fig. 2a,b ), suggesting that invasion-blocking mAbs act independently of erythrocyte binding. To further determine the epitope specificity, four N-terminal overlapping fragments (N1–N4) derived from RII-3 were expressed as recombinant proteins and screened using the mAbs ( Supplementary Fig. S3 ). The size of each fragment was confirmed using anti-His-tag mAbs ( Supplementary Fig. S3f ). None of the PfRH1 mAbs recognizes N1, whereas C2, C41 and C49 recognize N4 only. C50 is able to detect N2, N3 and N4 ( Supplementary Fig. S3b–e ), suggesting that C50 binds to a different epitope from that of C2, C41 or C49. On the basis of the western blot results, we further synthesized six overlapping peptides ( Supplementary Fig. S3g ). The inhibitory mAbs C41 and C49, as well as the non-inhibitory mAb C2, recognize the same 15-mer peptide, whereas another non-inhibitory mAb C50 recognizes a different peptide ( Supplementary Fig. S3h ). It is somewhat surprising that the non-inhibitory and inhibitory mAbs recognize the same peptide; however, as an epitope is 5–8 amino-acid long, it is possible that multiple distinct epitopes lie within the same peptide. In fact, previous studies have shown that mAbs against epitopes that are very close to each other exhibit different effects on cellular or biological functions [20] , [21] , [22] . 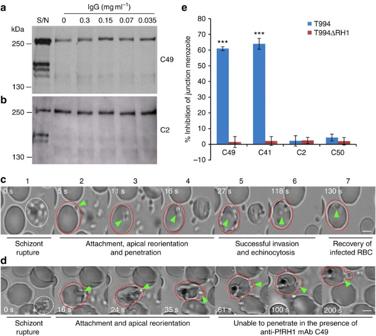Figure 2: Anti-PfRH1 mAbs inhibit invasion before junction formation. (a,b) Erythrocyte binding assays of T994 parasite culture supernatants using the C49 (a) and C2 (b) mAbs. Neither C49 nor C2 (0.035–0.3 mg ml−1) was able to inhibit the erythrocyte binding of PfRH1. T994 parasite culture supernatants (S/N) were used as a quality control. Molecular sizes are indicated on the left (in kDa). (c,d) Snapshots taken from time-lapse live movie microscopy of invasion of W2mef by merozoites in the absence (c) or presence (d) of C49 mAb. Time-elapsed post schizont rupture is indicated in each snapshot in seconds (sec, white). A white dotted circle indicates a rupturing schizont. Green arrows point to merozoites. A red dotted circle around an erythrocyte is added to help follow the infection. Scale bars=5 μM. (c) In the absence of mAb, the merozoite released from a mature schizont (white cycle) attaches, apically reorients and penetrates into an uninfected erythrocyte. Following successful invasion, deformation of infected erythrocytes occurs (echinocytosis) and by 2 min the erythrocytes recover back to its normal shape. (d) In the presence of C49, the merozoite released from a mature schizont attaches and apically reorients, but it is unable to penetrate the erythrocyte even after 3 min. Also seeSupplementary Movies 1,2. (e) Anti-PfRH1 inhibitory mAbs significantly reduce merozoite junction formation. T994 or T994ΔRH1 schizonts were pretreated with Cyto D and allowed to rupture in the absence or presence of anti-PfRH1 mAbs (0.2 mg ml−1). Junction-arrested merozoites were counted microscopically. Bar chart indicates the counting of junction-arrested merozoites with mAbs C2, C41, C49 and C50 in T994 and T994ΔRH1 compared with the arrested parasites in the absence of mAbs. Inhibitory mAbs C49 and C41 significantly blocked merozoite junction formation in T994. The error bar indicates the s.e.m.;n=3. ***P≤0.00014 by one-way ANOVA indicates the significant differences between the effects of inhibitory mAbs (C49 and C41) and those of non-inhibitory mAbs (C2 and C50). Figure 2: Anti-PfRH1 mAbs inhibit invasion before junction formation. ( a , b ) Erythrocyte binding assays of T994 parasite culture supernatants using the C49 ( a ) and C2 ( b ) mAbs. Neither C49 nor C2 (0.035–0.3 mg ml −1 ) was able to inhibit the erythrocyte binding of PfRH1. T994 parasite culture supernatants (S/N) were used as a quality control. Molecular sizes are indicated on the left (in kDa). ( c , d ) Snapshots taken from time-lapse live movie microscopy of invasion of W2mef by merozoites in the absence ( c ) or presence ( d ) of C49 mAb. Time-elapsed post schizont rupture is indicated in each snapshot in seconds (sec, white). A white dotted circle indicates a rupturing schizont. Green arrows point to merozoites. A red dotted circle around an erythrocyte is added to help follow the infection. Scale bars=5 μM. ( c ) In the absence of mAb, the merozoite released from a mature schizont (white cycle) attaches, apically reorients and penetrates into an uninfected erythrocyte. Following successful invasion, deformation of infected erythrocytes occurs (echinocytosis) and by 2 min the erythrocytes recover back to its normal shape. ( d ) In the presence of C49, the merozoite released from a mature schizont attaches and apically reorients, but it is unable to penetrate the erythrocyte even after 3 min. Also see Supplementary Movies 1,2 . ( e ) Anti-PfRH1 inhibitory mAbs significantly reduce merozoite junction formation. T994 or T994ΔRH1 schizonts were pretreated with Cyto D and allowed to rupture in the absence or presence of anti-PfRH1 mAbs (0.2 mg ml −1 ). Junction-arrested merozoites were counted microscopically. Bar chart indicates the counting of junction-arrested merozoites with mAbs C2, C41, C49 and C50 in T994 and T994ΔRH1 compared with the arrested parasites in the absence of mAbs. Inhibitory mAbs C49 and C41 significantly blocked merozoite junction formation in T994. The error bar indicates the s.e.m. ; n =3. *** P ≤0.00014 by one-way ANOVA indicates the significant differences between the effects of inhibitory mAbs (C49 and C41) and those of non-inhibitory mAbs (C2 and C50). Full size image Live video microscopy is a powerful tool to dissect merozoite invasion, and it has been effectively used to demonstrate the role of another merozoite invasion protein, PfAMA1, during merozoite re-orientation step in invasion [23] . Using time-lapse live video microscopy, we followed the process of merozoite invasion both in the presence and absence of invasion inhibitory antibodies ( Fig. 2c,d , Supplementary Fig. S4a,b and Supplementary Movies 1–7 ). We found that, in the absence of antibodies, newly released merozoites rapidly attach, reorient and invade erythrocytes ( Fig. 2c and Supplementary Movie 1 ). Immediately after invasion, the erythrocyte shrinks and echinocytosis occurs, with the infected erythrocyte recovering its shape within 2 min. Interestingly, in the presence of the invasion inhibitory antibody C49 ( Fig. 2d and Supplementary Movie 2,6 ) or C41 ( Supplementary Fig. S4a and Supplementary Movie 3,7 ), merozoites are able to attach and reorient themselves but are unable to penetrate the erythrocyte even after 3 min, despite extensive distortions of the erythrocyte being observed. In contrast, invasion similar to that seen in the absence of any antibody is observed in the presence of the non-inhibitory antibodies C2 ( Supplementary Fig. S4b and Supplementary Movie 4 ) or C50 ( Supplementary Movie 5 ). The inability of the merozoite to penetrate the erythrocyte despite reorientation and clear binding suggests that the inhibitory antibodies interfere with a subsequent step of the invasion process. Junction formation is known to be linked to the irreversible commitment of the merozoite to invasion, and recent studies have shown that PfRH1, PfRH2a/2b and PfRH5 localize at the tight junction, suggesting a specific role for the PfRH proteins during this part of the invasion process [6] , [24] , [25] , [26] . Therefore, to assess whether the inhibitory mAbs prevented junction formation, merozoites were arrested at the tight junction by treatment with cytochalasin D (Cyto D) [27] . Experiments were carried out in the absence and presence of PfRH1 mAbs, and junction-arrested merozoites were counted. Similar to the invasion inhibition assay, inhibitory mAbs C49 and C41 significantly reduce junction-arrested merozoites as compared with C2 and C50 in both T994 and W2mef ( Fig. 2e , Supplementary Table S1 and Supplementary Fig. S4c ). In contrast, no effect is seen in T994ΔRH1 and W2mef/NM, in line with PfRH1 not having a role in these parasites. Taken together, these data clearly demonstrate that inhibitory mAbs inhibit the invasion before junction formation and suggest that PfRH1 could have a key signalling role ahead of junction formation. PfRH1 inhibitory mAbs block Ca 2+ signalling during invasion Previous work has suggested that secretion of EBA175 from the micronemes onto the surface of the merozoite is a prerequisite for junction formation and is triggered by calcium (Ca 2+ ) release in the merozoite [28] . Here we carried out real-time measurement of Ca 2+ signalling in the presence/absence of Cyto D during merozoite invasion using freshly isolated free merozoites from T994 parasite. We found that Ca 2+ signal increases both in the presence and absence of Cyto D ( Fig. 3a , Supplementary Data 1–6 ), demonstrating that the signal originates before or at junction formation. This allowed us to further elucidate whether the invasion inhibitory mAbs targeting PfRH1 directly had an impact on Ca 2+ signalling. We observed that the cumulative intracellular Ca 2+ signal during merozoite invasion is significantly reduced in the presence of the inhibitory mAbs C41, as compared with the non-inhibitory mAbs C2 or no antibody control ( Fig. 3b , Supplementary Data 1–6 ). No antibody effect on Ca 2+ signalling is seen in T994ΔRH1 ( Fig. 3c , Supplementary Data 1–6 ). These results suggest that PfRH1 inhibitory mAbs inhibit invasion by blocking Ca 2+ signalling. Control experiments using the Ca 2+ ionophore A23187 and the Ca 2+ chelator BAPTA-AM showed that treatment of merozoites with A23187 leads to a significant increase in the Ca 2+ signal over time, whereas pretreatment with BAPTA-AM significantly reduces Ca 2+ signals ( Supplementary Fig. S5 , Supplementary Data 1–6 and Supplementary Table S2 ). Although the Ca 2+ signal observed during invasion assays is only derived from successfully invading merozoites, all viable merozoites are expected to give Ca 2+ signals after A23187 treatment, explaining the higher signal obtained (compare Fig. 3b with Supplementary Fig. S5 ). Importantly, functional C41 Fab fragments also block Ca 2+ signalling in T994 parasite during invasion ( Fig. 3d , Supplementary Data 1–6 ) as effectively as mAbs C41. This further confirms that the specific binding of inhibitory mAbs to PfRH1 is important for blocking Ca 2+ signalling. 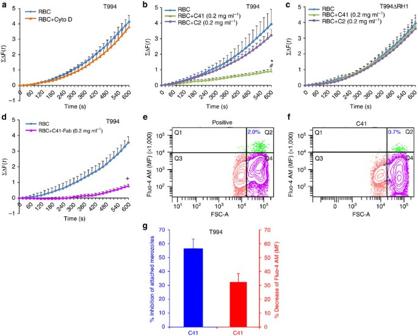Figure 3: Detection of cytosolic Ca2+levels during merozoite invasion. (a–d) Cytosolic Ca2+levels were detected using a fluorescence plate reader. (a) Preloaded T994 merozoites with Fluo-4AM were incubated with erythrocytes in the absence (RBC) or presence of Cyto D (RBC+Cyto D). (b,c) Preloaded T994 (b) or T994ΔRH1 (c) merozoites were incubated with erythrocytes in the absence (RBC) and presence of either C41 (RBC+C41 (0.2 mg ml−1)) or C2 (RBC+C2 (0.2 mg ml−1)). (d) Preloaded T994 merozoites were incubated with erythrocytes in the absence (RBC) or presence of mAb C41 Fab fragment (C41 Fab (0.2 mg ml−1)). The cumulative changes of Ca2+levels (≤ΔF (t)) in merozoites over 600 s were summed up and plotted against time (s). Experimental data were presented as the mean±s.e.m.;n=3. *P≤0.0001 by one-way ANOVA, indicating that C41 successfully blocked the Ca2+signalling in T994 when compared with the absence of C41.#P≤0.0001 by one-way ANOVA, indicating that C41 successfully blocked the Ca2+signalling in T994 when compared with the presence of C2.+P≤0.0001 by one-way ANOVA, indicating that C41 Fab fragment significantly inhibited the Ca2+signalling in T994, when compared with the absence of C41 Fab fragment. (e–g) Cytosolic Ca2+levels detected by flow cytometry. Representative FACS contour plots (e,f) were gated by size (FSC-A) versus mean fluorescence (MF) of Fluo-4 AM of merozoite (DAPI (+)) incubated with erythrocytes in the absence (e, Positive) or presence of C41 (f, C41). Vertical gating is to separate the free merozoites with low FSC from the RBC-attached merozoites with high FSC, whereas horizontal gating is to differentiate intercellular Ca2+levels. Q1 (green) represents free merozoites with Fluo-4 AM signals. Q2 (green) represents invading merozoites with increasing Fluo-4 AM signals. The number (blue) in Q2 represents % population of attached merozoites. Q3 (peach) represents free merozoites with no signal. Q4 (pink) represents attached merozoites with no signal. (g) Statistical analysis of the effect of C41 on Ca2+signalling during T994 merozoite invasion by FACS. C41 was able to reduce the number of invading merozoites to 56.6% (blue) and to decrease the overall Ca2+level to 32.42% (red) during invasion, as compared with that in the absence of C41. Experimental data are presented as the mean±s.e.m.;n=3. Figure 3: Detection of cytosolic Ca 2+ levels during merozoite invasion. ( a – d ) Cytosolic Ca 2+ levels were detected using a fluorescence plate reader. ( a ) Preloaded T994 merozoites with Fluo-4AM were incubated with erythrocytes in the absence (RBC) or presence of Cyto D (RBC+Cyto D). ( b , c ) Preloaded T994 ( b ) or T994ΔRH1 ( c ) merozoites were incubated with erythrocytes in the absence (RBC) and presence of either C41 (RBC+C41 (0.2 mg ml −1 )) or C2 (RBC+C2 (0.2 mg ml −1 )). ( d ) Preloaded T994 merozoites were incubated with erythrocytes in the absence (RBC) or presence of mAb C41 Fab fragment (C41 Fab (0.2 mg ml −1 )). The cumulative changes of Ca 2+ levels (≤ΔF (t)) in merozoites over 600 s were summed up and plotted against time (s). Experimental data were presented as the mean±s.e.m. ; n =3. * P ≤0.0001 by one-way ANOVA, indicating that C41 successfully blocked the Ca 2+ signalling in T994 when compared with the absence of C41. # P ≤0.0001 by one-way ANOVA, indicating that C41 successfully blocked the Ca 2+ signalling in T994 when compared with the presence of C2. + P ≤0.0001 by one-way ANOVA, indicating that C41 Fab fragment significantly inhibited the Ca 2+ signalling in T994, when compared with the absence of C41 Fab fragment. ( e – g ) Cytosolic Ca 2+ levels detected by flow cytometry. Representative FACS contour plots ( e , f ) were gated by size (FSC-A) versus mean fluorescence (MF) of Fluo-4 AM of merozoite (DAPI (+)) incubated with erythrocytes in the absence ( e , Positive) or presence of C41 ( f , C41). Vertical gating is to separate the free merozoites with low FSC from the RBC-attached merozoites with high FSC, whereas horizontal gating is to differentiate intercellular Ca 2+ levels. Q1 (green) represents free merozoites with Fluo-4 AM signals. Q2 (green) represents invading merozoites with increasing Fluo-4 AM signals. The number (blue) in Q2 represents % population of attached merozoites. Q3 (peach) represents free merozoites with no signal. Q4 (pink) represents attached merozoites with no signal. ( g ) Statistical analysis of the effect of C41 on Ca 2+ signalling during T994 merozoite invasion by FACS. C41 was able to reduce the number of invading merozoites to 56.6% (blue) and to decrease the overall Ca 2+ level to 32.42% (red) during invasion, as compared with that in the absence of C41. Experimental data are presented as the mean±s.e.m. ; n =3. Full size image We performed similar experiments using flow cytometry to measure Ca 2+ levels during invasion of fresh erythrocytes by free merozoites in the presence of Cyto D, as well as in the presence/absence of inhibitory mAbs. Invading merozoites will be arrested by Cyto D after junction formation, whereas merozoites in the presence of inhibitory antibodies will either detach or remain attached to the RBC without forming a junction. On the basis of these criteria, there are two distinct populations: free merozoites and RBC-bound merozoites. Staining for DAPI (+) events identifies all merozoites, whereas gating for size enables us to distinguish between free and RBC-bound merozoites ( Fig. 3e,f ). An inhibitory antibody C41 can reduce the number of invading merozoites to 56.6% ( Fig. 3g -blue) and decrease the overall Ca 2+ level to 32.42% ( Fig. 3g -red) during invasion, when compared with the absence of inhibitory mAbs. This result is consistent with our previous conclusion, supporting the accessibility and reproducibility of real-time measurement of Ca 2+ signalling by using a fluorescence plate reader. Taken together, these results strongly support the conclusion that PfRH1 has a direct or indirect role in the regulation of Ca 2+ signalling during invasion. Hence, we propose that binding of the mAbs to PfRH1 directly inhibits a signal to trigger Ca 2+ signal, or it has an indirect effect by preventing the recruitment of other proteins important for the initiation of the signal. Merozoite viability To ensure that the observed Ca 2+ signal was indeed due to merozoite invasion, each merozoite preparation in parallel to Ca 2+ signalling studies was assessed for their ability to invade fresh erythrocytes. T994 and T994ΔRH1 merozoites from each preparation successfully invade erythrocytes, and T994 invasion is successfully inhibited by C41 but not C2. In contrast, none of the antibodies has any impact on invasion in the case of T994ΔRH1 ( Supplementary Table S3 ). Importantly, there is a clear correlation ( R 2 =0.836) between invasion and Ca 2+ signal, with low invasion (due to antibody blocking) leading to low Ca 2+ signal ( Fig. 4a ). In addition, we followed the kinetics of merozoite invasion using heparin treatment [29] and observed that almost 75% of isolated merozoites invade erythrocytes in a linear manner ( R 2 =0.991) over the first 10 min ( Fig. 4b ), which is in line with time-dependent Ca 2+ data. Only a small proportion (25%) of the total invading merozoites have not invaded within 10 min, confirming that the observed increase in Ca 2+ signal was contributed by the majority proportion of invading merozoites over the first 10 min. Taken together, these data clearly indicate that viable invasion-competent merozoites contribute to the signals. 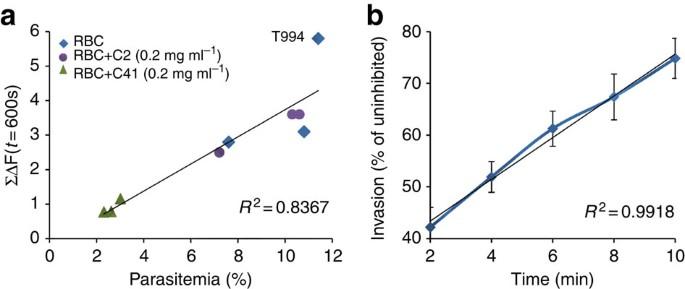Figure 4: Correlation between invasion and Ca2+signal. (a) T994 merozoites isolated from each Ca2+measurement experiment (Fig. 3b) were also used in parallel to test invasion (Supplementary Table S3). The percentage of invasion (Parasitemia (%), horizontal axis) is plotted against the Ca2+signals att=600 s (≤ΔF (t=600 s), vertical axis) (Fig. 3b). Blue diamonds represent merozoites incubated with erythrocytes in the absence of mAbs (RBC). Green triangles represent merozoites incubated with erythrocytes in the presence of inhibitory mAb C41 (RBC+C41 (0.2 mg ml−1)). Purple circles represent merozoites incubated with erythrocytes in the presence of non-inhibitory mAb C2 (RBC+C2 (0.2 mg ml−1)). TheR-square (R2) with value of 0.836 indicates strong correlation between invasion and Ca2+signalling. (b) Merozoite invasion kinetics assay under heparin treatment. Freshly isolated T994 merozoites were allowed to invade erythrocytes followed by treatment with heparin (200 μg ml−1) at different time points (2–10 min with 2 min interval) to inhibit invasion. After the final time point, cultures were incubated for 40 h, and resulting parasitemias were analysed by flow cytometry. The proportion of merozoites that have invaded with increasing time is shown as % of maximum invasion obtained in uninhibited culture. The rate of merozoite invasion over time is linear (R2=0.991). Experimental data are presented as the mean±s.e.m.;n=3. Figure 4: Correlation between invasion and Ca 2+ signal. ( a ) T994 merozoites isolated from each Ca 2+ measurement experiment ( Fig. 3b ) were also used in parallel to test invasion ( Supplementary Table S3 ). The percentage of invasion (Parasitemia (%), horizontal axis) is plotted against the Ca 2+ signals at t =600 s (≤ΔF ( t =600 s), vertical axis) ( Fig. 3b ). Blue diamonds represent merozoites incubated with erythrocytes in the absence of mAbs (RBC). Green triangles represent merozoites incubated with erythrocytes in the presence of inhibitory mAb C41 (RBC+C41 (0.2 mg ml −1 )). Purple circles represent merozoites incubated with erythrocytes in the presence of non-inhibitory mAb C2 (RBC+C2 (0.2 mg ml −1 )). The R -square ( R 2 ) with value of 0.836 indicates strong correlation between invasion and Ca 2+ signalling. ( b ) Merozoite invasion kinetics assay under heparin treatment. Freshly isolated T994 merozoites were allowed to invade erythrocytes followed by treatment with heparin (200 μg ml −1 ) at different time points (2–10 min with 2 min interval) to inhibit invasion. After the final time point, cultures were incubated for 40 h, and resulting parasitemias were analysed by flow cytometry. The proportion of merozoites that have invaded with increasing time is shown as % of maximum invasion obtained in uninhibited culture. The rate of merozoite invasion over time is linear ( R 2 =0.991). Experimental data are presented as the mean±s.e.m. ; n =3. Full size image An EBA175 inhibitory mAb has no effect on Ca 2+ signalling In line with published data, our results indicate that PfRH1 has a direct role in Ca 2+ release, which then triggers microneme and EBA175 secretion. If this is indeed correct, it would be expected that blocking EBA175 function and thereby junction formation would have no impact on Ca 2+ signalling. To investigate this further, we used the invasion-blocking mAb R215, which targets EBA175 region II (ref. 30 ). As previously described, mAb R215 is able to dose-dependently block invasion, with maximum inhibition around 47.7% ±1.11 at 0.25 mg ml −1 ( Fig. 5a ) [30] . However, this antibody has no effect on intracellular Ca 2+ signalling during invasion ( Fig. 5b , Supplementary Data 1–6 ). This result confirms that invasion-blocking antibodies targeting EBA175 act after Ca 2+ signalling, whereas those targeting PfRH1 act before Ca 2+ signalling, and clearly highlights the different roles that are performed by PfRH1 and EBA175. 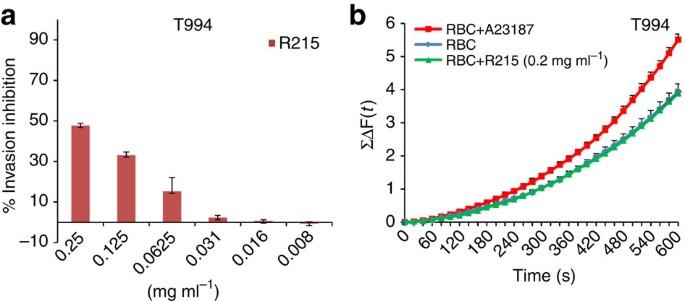Figure 5: The R215 mAb against EBA175 region II inhibits invasion but not Ca2+signalling. (a) Invasion inhibition assay using anti-EBA175 mAb R215 in T994 parasites. Bar charts show invasion inhibition of different concentrations (0.25–0.008 mg ml−1) of the EBA175-specific mAb R215 in T994. Bar charts show mean±s.e.m.;n=3. (b) Cytosolic Ca2+levels were detected by using a fluorescence plate reader. Preloaded T994 merozoites with Fluo-4AM were incubated with erythrocytes in the absence (RBC) or presence of R215 (RBC+R215 (0.2 mg ml−1)). Ca2+ionophore A23187 (RBC+A23187) was used as positive control. Changes in cytosolic Ca2+levels during merozoite invasion were assessed over time using a fluorescence plate reader. ≤ΔF(t) that reflects the total changes of cytosolic Ca2+levels in merozoites were plotted against time (s). Experimental data were presented as the mean±s.e.m.;n=3. Figure 5: The R215 mAb against EBA175 region II inhibits invasion but not Ca 2+ signalling. ( a ) Invasion inhibition assay using anti-EBA175 mAb R215 in T994 parasites. Bar charts show invasion inhibition of different concentrations (0.25–0.008 mg ml −1 ) of the EBA175-specific mAb R215 in T994. Bar charts show mean±s.e.m. ; n =3. ( b ) Cytosolic Ca 2+ levels were detected by using a fluorescence plate reader. Preloaded T994 merozoites with Fluo-4AM were incubated with erythrocytes in the absence (RBC) or presence of R215 (RBC+R215 (0.2 mg ml −1 )). Ca 2+ ionophore A23187 (RBC+A23187) was used as positive control. Changes in cytosolic Ca 2+ levels during merozoite invasion were assessed over time using a fluorescence plate reader. ≤ΔF(t) that reflects the total changes of cytosolic Ca 2+ levels in merozoites were plotted against time (s). Experimental data were presented as the mean±s.e.m. ; n =3. Full size image PfRH1 inhibitory mAbs block EBA175 expression To investigate whether the inhibition of Ca 2+ signalling by PfRH1 inhibitory mAbs has a downstream effect on the surface expression of EBA175, we assessed the translocation of EBA175 onto the merozoite surface. Merozoites arrested by Cyto D during erythrocyte invasion in the presence/absence of invasion inhibitory mAbs were surface stained with either antibodies against EBA175 or the merozoite surface marker MSP1. Surface expression of EBA175 was observed under fluorescence microscopy or measured under the fluorescence plate reader. Microneme protein EBA175 of impermeabilized merozoites will not be stained unless they are translocated to the surface of merozoites. Immunofluorescence assays clearly showed that the invasion inhibitory antibody C41 blocks surface expression of EBA175 in T994 ( Fig. 6a lower panel), whereas it has no effect on T994ΔRH1 parasites ( Fig. 6b lower panel). In the absence of C41, EBA175 is expressed on the surface of both T994 and T994ΔRH1 (upper panels of Fig. 6a,b ). In contrast, the inhibitory antibody has no effect on the detection of MSP1 on the surface of merozoites ( Fig. 6c,d ). Quantification of the overall impact of EBA175 surface expression in the parasite population was assessed using a fluorescent plate reader. In T994, overall EBA175 surface expression is reduced by >35% by the inhibitory antibody C41, whereas no impact is seen in T994ΔRH1 or on the surface expression of MSP1 ( Fig. 6e and Supplementary Table S4 ). Streptolysin O (SLO) is often used to selectively permeabilize the plasma membrane of P. falciparum -infected erythrocytes by forming stable proteinaceous pores without altering the orientation of membrane proteins [31] . Permeabilization of T994 merozoites with SLO before staining with EBA175 antibody showed no difference in overall EBA175 expression (internal and surface) between free and junction-arrested merozoites in C41-treated cultures as compared with the control. This result was confirmed by performing immunofluorescence assays and by measurement using the fluorescent plate reader ( Supplementary Fig. S6 and Supplementary Table S5 ). To further determine whether SLO could effectively permeabilize merozoite membrane to distinguish protein expression internally or on the surface, nucleoporin 100 (Nup 100; a nuclear periphery marker) and histone marker H3K9ac were used [32] . In merozoite permeabilized with SLO, Nup 100 localizes in the nuclear periphery outside the DAPI-stained area, whereas H3K9ac tends to co-localize with DAPI-stained area ( Supplementary Fig. S7a,b ). No staining was found in impermeabilized merozoites ( Supplementary Fig. S7c,d ). Taken together, these data confirm that C41 blocks EBA175 surface expression on merozoites during invasion. 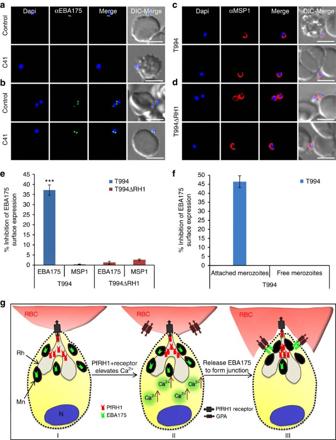Figure 6: Effect of anti-PfRH1 inhibitory mAbs on merozoite surface expression of EBA175 during invasion. (a–d) Surface expression of EBA175 and MSP1 on T994 and T994ΔRH1 was detected by immunofluorescence assays. Isolated T994 (a,c) or T994ΔRH1 (b,d) merozoites were directly incubated with erythrocytes containing 4 μM Cyto D in the absence (Control) and presence (C41) of C41 (0.2 mg ml−1) before analysis of expression of EBA175 and MSP1 at the junction. Both differential interference contrast (DIC) and fluorescence images were captured. Nuclear DNA was counterstained with DAPI (blue). EBA175 is shown in green, whereas MSP1 is shown in red. Fluorescence images, merged fluorescence images (DAPI and green or DAPI with red) and merged fluorescence images with DIC images are shown. Scale bars=10 μM. (e) EBA175 surface expression on merozoites was detected by using a fluorescence plate reader. Surface expression of EBA175 and MSP1 on merozoite in the presence of C41 was compared with their controls. Experimental data are presented as the mean±s.e.m.;n=3. ***P≤0.000025 by one-way ANOVA, indicating that C41 significantly decreases the surface expression of EBA175 in T994. (f) T994 merozoite EBA175 surface expression was also detected by flow cytometry during invasion (detail shown inSupplementary Fig. S8). Statistical analysis of the effect of C41 on merozoite EBA175 surface expression is shown. Merozoite attached to RBCs surface expression of EBA175 in the presence of C41 was compared with its positive control. Experimental data are presented as the mean±s.e.m.;n=4. (g) Schematic diagram of Ca2+signalling in junction formation during erythrocyte invasion. After the merozoite initially attaches to the erythrocyte (RBC) and reorients itself, PfRH1 released from rhoptry (Rh) is responsible for sensing the apical end interaction (I). The binding of PfRH1 to its receptor triggers an increase of intracellular Ca2+(II). Rise in cytosolic Ca2+levels results in release of microneme (Mn) proteins such as EBA175 to bind to glycophorin A (GPA), which leads to tight junction formation (III). Figure 6: Effect of anti-PfRH1 inhibitory mAbs on merozoite surface expression of EBA175 during invasion. ( a – d ) Surface expression of EBA175 and MSP1 on T994 and T994ΔRH1 was detected by immunofluorescence assays. Isolated T994 ( a , c ) or T994ΔRH1 ( b , d ) merozoites were directly incubated with erythrocytes containing 4 μM Cyto D in the absence (Control) and presence (C41) of C41 (0.2 mg ml −1 ) before analysis of expression of EBA175 and MSP1 at the junction. Both differential interference contrast (DIC) and fluorescence images were captured. Nuclear DNA was counterstained with DAPI (blue). EBA175 is shown in green, whereas MSP1 is shown in red. Fluorescence images, merged fluorescence images (DAPI and green or DAPI with red) and merged fluorescence images with DIC images are shown. Scale bars=10 μM. ( e ) EBA175 surface expression on merozoites was detected by using a fluorescence plate reader. Surface expression of EBA175 and MSP1 on merozoite in the presence of C41 was compared with their controls. Experimental data are presented as the mean±s.e.m. ; n =3. *** P ≤0.000025 by one-way ANOVA, indicating that C41 significantly decreases the surface expression of EBA175 in T994. ( f ) T994 merozoite EBA175 surface expression was also detected by flow cytometry during invasion (detail shown in Supplementary Fig. S8 ). Statistical analysis of the effect of C41 on merozoite EBA175 surface expression is shown. Merozoite attached to RBCs surface expression of EBA175 in the presence of C41 was compared with its positive control. Experimental data are presented as the mean±s.e.m. ; n =4. ( g ) Schematic diagram of Ca 2+ signalling in junction formation during erythrocyte invasion. After the merozoite initially attaches to the erythrocyte (RBC) and reorients itself, PfRH1 released from rhoptry (Rh) is responsible for sensing the apical end interaction (I). The binding of PfRH1 to its receptor triggers an increase of intracellular Ca 2+ (II). Rise in cytosolic Ca 2+ levels results in release of microneme (Mn) proteins such as EBA175 to bind to glycophorin A (GPA), which leads to tight junction formation (III). Full size image We provide additional support for the surface expression of EBA175 on junction-arrested T994 merozoites using flow cytometry. Isolated merozoites were allowed to invade fresh erythrocytes in the presence of Cyto D as well as in the presence/absence of inhibitory mAbs. In addition, labelling for EBA175 surface expression with anti-EBA175 antibodies allowed us to identify the population of free and arrested merozoites that express EBA175 on their surface. Analysis of ~5,000 DAPI (+) merozoites showed that, in the absence of inhibitory antibodies, free merozoites make up 47.1% of population, of which 0.2% show EBA175 staining. In contrast, 40.7% of the 52.9% RBC-bound merozoites show EBA175 staining. In the presence of invasion inhibitory antibodies, free merozoites make up 52% of population, of which 0.5% are EBA175 positive, whereas only 17% of the 47.8% RBC-bound merozoites are EBA175 positive ( Supplementary Fig. S8 ). The data show that there is an ~45% inhibition of EBA175 surface expression in RBC-bound merozoites in the presence of the invasion inhibitory antibody ( Fig. 6f ), in line with the data obtained using the fluorescence plate reader ( Fig. 6e ). In addition, these results show that free merozoites hardly express EBA175 on the surface; furthermore, it also shows that in the absence of invasion inhibitory antibodies more RBC-attached merozoites are expressing EBA175, in line with them having formed a junction. Taken together, our data provide the first evidence that PfRH1 has a crucial role in triggering intracellular Ca 2+ signal, which then leads to the subsequent release of EBA175 to form tight junction. Ca 2+ is a second messenger in eukaryotic cell signalling and is typically released from intracellular stores in response to an external stimulus (chemical, electrical or mechanical) that triggers a signalling cascade, which leads to a rise in cytoplasmic-free calcium [33] . Apical secretion of micronemal and rhoptry proteins has been observed upon contact of the apicomplexan parasite Toxoplasma gondii [34] , [35] as well as P. falciparum [36] , [37] with their host cells, thereby mediating invasion. In T. gondii increased intracellular Ca 2+ has been shown to trigger both microneme protein secretion as well as parasite egress from host cell [35] , [38] , and recently it has been shown that a rise in cytosolic Ca 2+ because of the Ca 2+ ionophore A23187 triggers secretion of microneme proteins such as EBA175 to the merozoite surface [28] . The precise signalling mechanisms that lead to the release of invasion proteins in a coordinated manner during invasion are not clear. Recent work by Singh et al. has shown that increase in the intracellular Ca 2+ is the key step leading to the release of EBA175 from the microneme. EBA175 binding to its glycophorin receptor subsequently leads to the release of rhoptry proteins CLAG3.1 and PfRH2b. This is in line with our findings that PfRH1-induced Ca 2+ signalling triggers EBA175 release. Previous work has shown that RH proteins appear to be located at the rhoptry neck, and our data would indicate that this enables at least some of the RHs to mediate the initial interactions with the erythrocyte thereby triggering Ca 2+ release and microneme discharge. The bulk of the rhoptry content, including the majority of RH, is discharged only after microneme release. It will now be interesting to establish any additional roles for RHs beyond the initial sensing. In the study by Singh et al. , Ca 2+ release is triggered by changing the concentration of K + in the buffer from a high to a low to reflect difference in the concentration of K + inside erythrocyte as compared with the blood plasma. In contrast, in our study, merozoites are kept in normal growth media that require PfRH1 engagement with erythrocytes to trigger Ca 2+ release. In future, it is desirable to further address the effect of K + level changes compared with PfRH1-mediated changes for eliciting Ca 2+ level increases. This could determine whether the K + -mediated signalling is upstream or independent of the PfRH1-mediated signalling during invasion. The relative importance of the two mechanisms in vivo also needs to be resolved. On the basis of our data, we hypothesize that the complex invasion process begins with a relatively small amount of PfRH1 exposed at the rhoptry duct interacting with its receptor on the erythrocyte surface, thereby either directly or indirectly activating a signalling cascade that leads to the release of intracellular Ca 2+ stores, followed by triggering microneme and rhoptry discharge and junction formation ( Fig. 6g ). This is consistent with a recent finding showing that Ca 2+ -mediated microneme discharge is important for invasion in both T. gondii and P. falciparum [39] . Our results also demonstrate a function for RHs that is independent of rhoptry discharge and occurs after microneme secretion, possibly indicating that RHs are moved to an active site ahead of the release of the rest of the rhoptry content. In future, it will now be important to further determine the mechanism by which the RH-mediated signal is passed to the merozoite to trigger Ca 2+ release. Overall, our results provide new insights on the finely regulated signalling cascade that is required to ensure successful invasion of the merozoite and to open up a path for the analysis of signalling pathways involved in regulated secretion of apical organelles during invasion. Together this will provide us with a better understanding of the signalling mechanisms important in merozoite invasion and how these processes might be a new target for malaria intervention. P. falciparum strains and culture P. falciparum parasite lines T994, W2mef (MR4) and T994ΔRH1 (ref. 40 ) were cultured in fresh erythrocytes from healthy human donors (after obtaining informed consent) and RPMI supplemented with 5% albumax (Invitrogen) [41] . W2mef parasites were allowed to grow in erythrocytes treated with 10 mU ml −1 neuraminidase (Nm; Roche). After 2–3 weeks, the W2mef parasite adapts and grows in neuraminidase-treated erythrocytes (sialic acid independent) [7] , [26] . This switched parasite was named W2mef/NM parasite. PfRH1 monoclonal antibodies generation and purification PfRH1 hybridoma cells were developed by BioGenes (Germany) using purified soluble recombinant protein PfRH1-RII-3 (ref. 7 ). Positively selected hybridoma cells were cultured in 2% FBS-DMEM (Invitrogen). Purification of PfRH1 mAbs IgG from cell culture medium was carried out by using standard purification procedures (HiTrap Protein G HP, GE healthcare). Monoclonal antibody C41 Fab fragment was generated and purified by using standard procedures (Pierce Fab Micro Preparation Kit, Thermo Scientific). The authenticity of the Fab fragment was confirmed by 12% SDS-PAGE (Bio-Rad) followed by coomassie blue staining (Sigma), which yielded one band of ~50 kDa under nonreducing conditions. Western blot of parasite extracts and culture supernatants Parasite culture was synchronized at the ring stage with 5% D -sorbitol (Sigma) and cultured to mature schizont stages [42] , [43] . Tightly synchronized late schizonts were purified using 68% Percoll gradient centrifugation [44] . Merozoites were purified from schizont extract by filtration under nitrogen cavitation [45] , [46] , [47] , [48] . Schizonts and merozoite extracts were washed twice with PBS, lysed directly into sample buffer and frozen and thawed three times, followed by separation on 12% SDS-PAGE. Mouse mAb g12 (1:1,000, MR4) [49] was used as a loading control for merozoite extracts, whereas rabbit α-actin polyclonal antibodies (1:1,000, Sigma) were used for schizont extracts. To make parasite culture supernatant, purified schizonts were allowed to grow in the absence of RBC at 37 °C with shaking. Cells were collected by centrifugation after 16 h, and supernatants were either stored in aliquots at −80 °C or directly separated on 6% SDS-PAGE. Micronemal marker EBA175-specific antibody [50] (1:5,000, MR4) was a loading control for parasite culture supernatant. Following electrophoresis, gels were transferred onto nitrocellulose membranes (0.2 μm) (Bio-Rad). Specific proteins were detected by using PfRH1 mAbs (1:5,000), followed by HRP-linked secondary antibodies (1:10,000) and enhanced chemiluminescence (GE healthcare). Invasion inhibition assay Synchronized late-stage schizonts were purified, and 160 μl of parasite suspension was added in duplicate in a 96-well flat bottom microtitre plate containing PfRH1 mAbs (0.008–0.5 mg ml −1 ), purified C41 Fab fragment (0.008–0.5 mg ml −1 ) or EBA175 mAb R215 (0.008–0.25 mg ml −1 ), respectively. A total of 1,000 erythrocytes were scored for presence of rings on Giemsa-stained smears after 24 h for reinvasion. Invasion (Inv) was assessed as (%) parasitemia. (%) Parasitemia=(total number of ring-infected RBCs/total number of RBCs) × 100. Invasion in the presence of mAbs was compared with positive controls of invasion of the same parasite lines in normal complete RPMI. Invasion inhibition efficiencies were determined as follows: (%) inhibition efficiency=(1−Inv(mAbs) dilu /Inv(positive)) × 100. Data shown are from three biological replicates. Each biological replicate has two technical replicates. Experimental data are presented as the mean±s.e.m. Erythrocyte binding assays Hundred microliters of T994 parasite culture supernatant was incubated with 100 μl of packed normal erythrocytes in the presence of PfRH1 mAbs (at final concentration ranging from 0.3 down to 0.035 mg ml −1 ) at 37 °C for 1 h [7] , [26] . Junction merozoite blocking assay Merozoites were arrested in the erythrocyte junction by treatment with cytochalasin D (Cyto D) (Sigma) [26] , [27] . Purified late-stage schizont parasites were added to the completed RPMI containing fresh erythrocytes in 96-well plates. Cyto D was added to the final concentration of 0.1 μM. PfRH1 mAbs were also present at 0.2 mg ml −1 concentration if required. After 8 h incubation, Giemsa (Sigma)-stained smears were prepared for counting merozoites arrested at junction formation by using light microscopy. A total of 1,000 erythrocytes were scored. The number of junction-arrested merozoites in the presence of mAbs was compared with that in a positive control of the same parasite. Junction merozoite inhibition efficiencies were determined as follows: % inhibition of junction merozoite=(1−total number of junction merozoites (mAbs)/total number of junction merozoites (positive control)) × 100. Data shown are from three biological replicates. Each biological replicate has two technical replicates. Experimental data are presented as the mean±s.e.m. Expression of four overlapping regions from RII-3 Four N-terminal overlapping fragments from RII-3 were amplified by PCR, expressed as His-tag recombinant proteins by BL21 (DE3) (Stratagene) [7] , named N1 (500–692 amino acid (aa)), N2 (500–726 aa), N3 (500–746 aa) and N4 (500–773 aa), followed by 12% SDS-PAGE and probed with mAbs C49, C41, C2 and C50, respectively (1:5,000). A mAb against 6X His-tag (αHis, 1:5,000, Clonetech) was used as loading control. For the PCR, the forward primer was 5′-GACCATATGTTACAAATAGTACAACAAAAACTTTTAGAAATC-3′ and the reverse primers were 5′-AACCTCGAGAGAAATAAGTTGAATCGTCTCATTATTTT-3′ (N1), 5′-AACCTCGAGGGATTTAAGAAGATTTTGGATGTTTT-3′ (N2), 5′-AACCTCGAGTTGTTTTAATATATATTTAGAAATTGTGTCTATGAA-3′ (N3), and 5′-AACCTCGAGGTTTTGTTCATTTTTTATTTCTTCAAGAT-3′ (N4). Peptide generation and epitope mapping of PfRH1 Peptide design was based on the mAbs recognition of four His-tag recombinant overlapping fragments derived from RII-3 by western blot ( Supplementary Fig. S3a–e ). All biotinylated overlapping synthetic peptides were synthesized by Peptide Synthesis Core facilities, SBS, NTU. The lyophilized peptides were dissolved in dimethyl sulfoxide (DMSO, Sigma). Peptide stocks were diluted in PBS+0.1% BSA to make up 2.5 μg ml −1 . The streptavidin-coated 96-well plate, pre-blocked with Superblock blocking buffer (Thermo Scientific), was washed three times with 200 μl wash buffer (25 mM Tris, 150 mM NaCl, pH 7.2, 0.1% BSA, 0.05% Tween 20). Hundred microliters of the peptide solution was added into each well of the streptavidin-coated plate and incubated for 2 h at room temperature (RT) with gentle shaking. After four washes, 100 μl of mAb (C49, C41, C2 or C50 in 25 mM Tris, 150 mM NaCl, pH 7.2, 0.1% BSA) at a concentration of 2.5 μg ml −1 was added into each well and incubated for 1 h at RT. The peptide was washed four times followed by the addition of 100 μl of HRP goat anti-mouse IgG (1:3,000; Biolegend). After six washes, 50 μl of 3,3′,5,5′-Tetramethylbenzidine (TMB) high sensitive substrate solution (Biolegend) was added into each well. The plates were incubated for 3–5 min before analysing by using a Benchmark PlusMicroplate Spectrophotometer (BioRad Laboratories Inc) at 370 nm. Live video microscopy For live video microscopy [23] , we used an Axiovert 200 M cell observer with a 37 °C chamber with a continuous supply of 5% CO 2 . Five to ten percentage of the late-schizont stage parasites were diluted at 1:100 in complete RPMI. Live video was performed using 35 mm glass bottom dishes. The video was captured in the presence or absence of PfRH1 mAbs (C2, C41, C49 and C50) at a final concentration of 0.2 mg ml −1 . AxioCam HRm camera and Axiovision software, or Cool SNAP camera and MetaMorph software, were used for image acquisition. The video files were prepared using Image J. Isolation of P. falciparum merozoites Purified P. falciparum schizonts were resuspended in warm complete RPMI and allowed to rupture and release merozoites over a period of 2 h at 37 °C. Cultures containing unruptured schizonts and released merozoites were centrifuged at 2,200 r.p.m. (942 g ) on an Eppendorf 5810R centrifuge for 3 min to separate released merozoites from unruptured schizonts and uninfected erythrocytes. Supernatants containing free merozoites were then centrifuged at 5,000 r.p.m. (4,500 g , Sigma 3K15) for 3 min to collect merozoites. The merozoites were immediately resuspended in warm complete RPMI medium for further studies. Viability assay of free merozoites Erythrocyte invasion assays were performed in parallel to assess the viability of isolated free merozoites tested for Ca 2+ measurement. After 24–30 h post-invasion, newly invaded ring-infected erythrocytes were scored by Giemsa (Sigma, USA) staining. Invasion rates were determined as (%) parasitemia. Data were shown from three biological replicates. Kinetics of merozoite invasion by heparin treatment To define the kinetics of merozoite invasion, the invasion inhibitor heparin was used to block merozoite invasion [29] . In brief, freshly isolated T994 merozoites were allowed to invade erythrocytes in the 96-well plate followed by addition of heparin (200 μg ml −1 ) at different time points (2–10 min with 2 min interval) to inhibit further invasion. After the final time point, cultures were incubated at 37 °C for 40 h. The plate was centrifuged at 2,200 r.p.m. (942 g ) for 3 min to separate free merozoites from uninfected and infected erythrocytes. The culture was washed with complete RPMI twice and stained with 40 nM 4′,6-diamidino-2-phenylindole (DAPI, Molecular Probes, USA). The resulting parasitemias were analysed by flow cytometry. The cells were first gated by size in SSC/FSC, followed by further gating in FSC-A/FSC-H to discriminate doublets from single cells. Uninfected erythrocytes were gated as baseline by DAPI fluorescence in FSC-A/DAPI-A. The proportion of merozoites that have invaded with increasing time is shown as % of maximum invasion obtained in uninhibited culture. Data shown were from three biological replicates. Experimental data were presented as the mean±s.e.m. ; n =3. Real-time Ca 2+ measurement in merozoites during invasion Fresh isolated merozoites were preloaded with 6 μM Fluo-4 AM (Invitrogen) in complete RPMI at 37 °C for 20 min. Preloaded merozoites were washed twice with warm complete RPMI and then immediately resuspended in fresh erythrocytes or in the presence of 4 μM Cyto D, C41, C2, C41 Fab fragment or EBA175 mAbs R215 at 0.2 mg ml −1 , or 10 μM Ca 2+ ionophore A23187 (Calbiochem, USA), or pretreated with 50 μM Ca 2+ chelator BAPTA-AM (Calbiochem, USA) followed by A23187 (ref. 28 ), and cultured in Greiner 96 Black Flat Bottom Polystyrol plates. Changes in cytosolic Ca 2+ levels during merozoite invasion were timely assessed using a fluorescence plate reader (Infinite M200; Tecan). Fluorescence intensity was measured for 600 s with excitation at 488 nm and emission at 530 nm by TECAN- i -control 1.8.20.0 software. The maximum increase of Ca 2+ green fluorescence (F) during a period of 600 s after the start of the stimulation was normalized to the fluorescence intensity before stimulation (F 0 ). Changes in cytosolic Ca 2+ levels (ΔF(t)) were expressed as changes in fluorescence intensity as a percentage of the starting fluorescence levels: ΔF(t)=(F−F 0 )/F 0 where F=fluorescence intensity (t), F 0 =starting fluorescence signal. The total changes of Ca 2+ levels (≤ΔF(t)) in merozoites along the 600 s were summed up and plotted against time (s). Data shown were from three biological replicates. Experimental data were presented as the mean±s.e.m. TECAN scanning was performed at 37 °C. Flow cytometry Ca 2+ measurement in merozoites during invasion Isolated T994 merozoites were preloaded with Fluo-4 AM as well as labelled with DAPI as described above, followed by incubation with fresh warm erythrocytes containing 4 μM Cyto D in the absence and presence of mAb C41 (0.2 mg ml −1 ). The culture was immediately processed using a BD LSR II flow cytometer (BD Biosciences). Merozoites that are invading will be arrested by Cyto D after junction formation, whereas merozoites in the presence of inhibitory antibodies will either detach or remain attached to the RBC without forming a junction. Each culture was excited with light at 488 and 355 nm, and fluorescence signal was detected with a 530/30 and 440/40 nm band pass filters. In each experiment, data were acquired for~20,000 DAPI (+) merozoites with the same settings for each condition. A histogram representing two distinct cell populations among these 20,000 cells indicates free merozoites and RBC-bound merozoites. Preloaded merozoites alone were measured as the baseline for detection of Fluo-4 AM signals. The cells were gated by FSC-A versus Fluo-4 AM mean fluorescence (MF). We observed the % parent population of attached merozoites with increasing Ca 2+ signal from the culture in the absence (positive) or presence of C41 (C41) and investigated the effect of C41 on signalling during invasion. Data were analysed by using BD FASCDiva software. (%) Inhibition of attached merozoites=(1−% parent population (C41)/% parent population (positive)) × 100. (%) Decrease of Fluo-4 AM mean fluorescence (MF)=(1−MF (C41)/MF (positive)) × 100. Data shown are from three biological replicates. Experimental data are presented as the mean±s.e.m. Measurement of intracellular Ca 2+ levels on free merozoites Merozoites preloaded with Fluo-4 AM as described above were immediately resuspended in complete RPMI only or treated with 10 μM A23187 for 15 min at 37 °C with or without pretreatment with 50 μM BAPTA-AM for 15 min at 37 °C (ref. 28 ). Changes in cytosolic Ca 2+ levels were assessed using flow cytometry. Preloaded merozoites in complete RPMI were measured as baselines. Merozoites were excited at 488 nm, and fluorescence signal is detected with a 530/30 nm band pass filter for periods of 2 min on BD LSR II (BD Biosciences). Merozoites were gated on the basis of their forward scatter (FSC) and side scatter (SSC). Data were evaluated by using dot plot of Fluo-4 AM mean fluorescence (MF) versus time using BD FACSDiva software to visualize the cytosolic Ca 2+ levels in merozoites. The effect of BAPTA-AM (MF BAPTA-AM ) on free merozoites Ca 2+ signalling was compared with that of A23187 (MF A23187 ). (%) Inhibition of BAPTA-AM=(1−(MF BAPTA-AM /MF A23187 )) × 100. Data shown are from three biological replicates. Experimental data are presented as the mean±s.e.m. Immunofluorescence assays and microscopy Synchronized late-stage schizonts were smeared and air-dried followed by fixation with acetone (Merck) for 5 min at RT. Smears were incubated with PfRH1 mAbs (1:800) and co-incubated with rabbit α-EBA175 (1:800) for 1 h in 3% BSA/PBS buffer, followed by three times for 5 min washes in 1 × PBS. They were then incubated with a mixture of Alex Flour 594 goat anti-mouse IgG (H+L) and Alex Flour 488 goat anti-rabbit IgG (H+L) secondary antibodies (1:1,000, respectively, Molecular Probe) for 1 h. Slides were washed in 1 × PBS for three times for 5 min. Slides were air-dried, mounting medium containing DAPI was applied (Vector laboratories), and the coverslips were sealed. The fluorescence images were captured using a LSM510 Confocal Microscope (Carl Zeiss). Immunofluorescence assay for merozoites Isolated T994 merozoites were incubated with or without streptolysin O (SLO, Sigma) [51] . The culture was washed three times with incomplete RPMI and then fixed with 1% p-formaldehyde (Sigma) for 45 min at RT followed by centrifugation at 5,000 r.p.m. (4,500 g , Sigma 3K15) for 3 min. After two washes, the culture was incubated with either rabbit α-Nucleoporin 100 (α-Nup 100, 1:500), a nuclear periphery marker, or rabbit α-acetyl-Histone H3 (Lys9) antibody (α-H3K9ac, 1:500, Millipore), a histone marker [32] for 45 min at 37 °C. The culture was washed three times in incomplete RPMI followed by incubation with Alex Flour 594 goat anti-rabbit IgG (H+L) (1:1,000) or Alex Flour 488 goat anti-rabbit IgG (H+L) (1:1,000) together with DAPI for 45 min at RT. The culture was washed three times and then applied to the slides. The images were captured by Nikon TE2000-U Inverted Fluorescence Microscopy. Detection of EBA175 on merozoite surface by fluorescence-based methods Isolated merozoites from T994 and T994ΔRH1 were incubated with fresh erythrocytes containing 4 μM Cyto D in the absence and presence of mAb C41 (0.2 mg ml −1 ) at 37 °C for 20 min followed by incubation with or without Streptolysin O (SLO, Sigma) [51] . The culture was washed three times with 1% BSA/PBS and then fixed with 1% p-formaldehyde (Sigma) for 45 min at RT followed by centrifugation at 5,000 r.p.m. (4,500 g , Sigma 3K15) for 3 min. After two washes, the culture was incubated with rabbit α-EBA175 (1:500) for 45 min at 37 °C. The culture was washed three times with incomplete RPMI followed by incubation with Alex Flour 488 goat anti-rabbit IgG (H+L) (1:1,000) together with DAPI for 45 min at RT. The culture was washed three times with incomplete RPMI. The culture was finally resuspended in 100 μl complete RPMI and transferred into Greiner 96 Black Flat Bottom Polystyrol plates for analysis by using a fluorescence plate reader using the program TECAN- i -control 1.8.20.0. The duplicated culture (except SLO treated culture) was also tested using rabbit α-MSP1 (1:1,000, MR4) followed by incubation with Alex Flour 594 goat anti-rabbit IgG (H+L) (1:1,000) together with DAPI. The samples were applied to the slides. The images were captured by Nikon TE2000-U Inverted Fluorescence Microscopy. To further confirm and quantify the effect of inhibitory mAbs C41 on the surface expression of EBA175, fluorescence intensity was also measured by using a fluorescence plate reader. Fluorescence signal of EBA175 (F EBA175 ) was excited at 488 nm and emitted at 519 nm, MSP1 surface staining (F MSP1 ) was excited at 590 nm and emitted at 617 nm and nuclear signal (F EBA175-DAPI or F MSP1-DAPI ) was excited at 375 nm and emitted at 461 nm. Fluorescence signal was normalized to nuclear DAPI signal as follows: EBA175 ratio=F EBA175 /F EBA175-DAPI and MSP1 ratio=F MSP1 /F MSP1-DAPI . Protein expression on merozoite surface in the presence of mAbs C41 was compared with its control of the same culture incubated in the absence of C41. Surface expression inhibition efficiencies were determined as follows: (%) inhibition of EBA175 surface expression=(1−EBA175 ratio (C41)/EBA175 ratio (control)) × 100 and (%) inhibition of MSP1 surface expression=(1−MSP1 ratio (C41)/MSP1 ratio (control)) × 100. Protein expression on merozoite permeabilized with SLO in the presence of mAbs C41 were compared with its control of the same culture in the absence of C41. EBA175 expression inhibition efficiencies were determined as follows: (%) inhibition of EBA175 expression=(1−EBA175 ratio (C41−SLO)/EBA175 ratio (control−SLO)) × 100. Data shown are from three biological replicates. Experimental data are presented as the mean±s.e.m. Detection of EBA175 on merozoite surface by flow cytometry The culture prepared for detection of EBA175 by fluorescence microscopy, mentioned above, was resuspended in complete RPMI and used for analysis by BD LSR II (BD Biosciences). In each experiment, data were acquired for 5,000 DAPI (+) merozoites with the same settings for each condition. A histogram representing two distinct cell populations among these 5,000 cells indicates free merozoites (Free Mero) and RBC-bound merozoites (Attached Mero+RBCs). We observed these two populations individually and investigated the effect of C41 on EBA175 surface expression in T994. Each culture was excited with light at 488 and 355 nm, and fluorescence signal was detected with 530/30 and 440/40 nm band pass filters. The cells were gated on the basis of their FSC and SSC. Data were analysed using BD FASCDiva software. Histograms showing logarithmic green fluorescence intensities (FITC-A) versus blue fluorescence intensities (DAPI-A) were plotted. For each experiment, fixed untreated cultures were stained only with FITC-conjugated anti-rabbit IgG to establish background staining and to set up a gate before calculating the percentage of FITC(+) merozoites (that is, those expressing EBA175 on their surface) in the parent population. EBA175 surface expression on junction-arrested merozoites in the presence of mAb C41 was compared with a positive control in the absence of C41. EBA175 surface expression inhibition efficiencies were determined as follows: (%) inhibition of EBA175 surface expression=(1−% parent population (C41)/% parent population (positive)) × 100. Data shown are from four biological replicates. Experimental data are presented as the mean±s.e.m. Statistical analysis Statistical comparison was done using one-way ANOVA as appropriate. The significance level was set at P <0.05. The P -value is provided for some individual experiments. Raw data of absolute measurement Ca 2+ signalling Absolute measurement raw data of all Ca 2+ signalling experiments have been provided in Supplementary Data 1–6 . How to cite this article: Gao, X. et al. Triggers of key calcium signals during erythrocyte invasion by Plasmodium falciparum . Nat. Commun. 4:2862 doi: 10.1038/ncomms3862 (2013).